Constructing minimal models for complex system dynamics One of the strengths of statistical physics is the ability to reduce macroscopic observations into microscopic models, offering a mechanistic description of a system’s dynamics. This paradigm, rooted in Boltzmann’s gas theory, has found applications from magnetic phenomena to subcellular processes and epidemic spreading. Yet, each of these advances were the result of decades of meticulous model building and validation, which are impossible to replicate in most complex biological, social or technological systems that lack accurate microscopic models. Here we develop a method to infer the microscopic dynamics of a complex system from observations of its response to external perturbations, allowing us to construct the most general class of nonlinear pairwise dynamics that are guaranteed to recover the observed behaviour. The result, which we test against both numerical and empirical data, is an effective dynamic model that can predict the system’s behaviour and provide crucial insights into its inner workings. Despite the marked advances in mapping social, biological and technological networks [1] , [2] , [3] , [4] , [5] , our ability to predict and manipulate their behaviour is currently limited due to the absence of accurate microscopic models of their interaction dynamics. Indeed, the observed behaviour of complex systems is governed by the interplay between their topology and their dynamics [6] , [7] , prompting us to develop reliable methodologies for the construction of dynamic models for complex systems. The problem is that unlike physical systems, where the interactions are described in terms of a set of fundamental rules, such as the laws of electromagnetism driving the microscopic interactions between particles, for most complex systems such rules remain to be discovered, limiting our ability to rely on a theoretical understanding of the system’s components when constructing the appropriate model. Here we develop a methodology to construct dynamic models directly from empirical observations, assuming minimal a priori knowledge about the system. Our goal is to directly translate these observations into a mechanistic model that accurately captures the interactions between the system’s components, ultimately providing the system’s equation of motion. Such models can provide both theoretical insights into the inner workings of the system and predictive power on its expected behaviour. Consider a complex system with N components (nodes), whose activities x i ( t ) ( i =1,…, N ) are driven by ordinary differential equations of the form Here M 0 ( x i ( t )) describes the self-dynamics of each component and M ( x i ( t ), x j ( t )) captures the impact of i ’s neighbour j on the state of i . The adjacency matrix, A ij , describes which components interact. With the appropriate choice of the nonlinear M 0 ( x i ( t )) and M ( x i ( t ), x j ( t )), equation (1) has been used before to describe the dynamics of a wide range of complex systems, like metabolic networks [8] , [9] , the spread of infectious disease on a social network [10] , [11] or interspecies interactions in ecological systems [12] , to mention only a few. Furthermore, for many biological [9] , [13] , [14] technological [15] or social [10] , [11] , [16] systems the interaction term factorizes as M ( x i ( t ), x j ( t ))= M 1 ( x i ( t )) M 2 ( x j ( t )), in which case the system’s dynamics is uniquely characterized by three independent functions, together defining the system’s model as a point in the model space ( Fig. 1a,b ). For systems of unknown microscopic dynamics, the challenge is to infer the appropriate model by identifying M 0 ( x ), M 1 ( x ) and M 2 ( x ) that accurately describe the system’s observable behaviour. (The treatment of more general systems, in which M ( x i , x j ) cannot be factorized, is discussed in Supplementary Note 5 ). 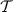Table 1 Observationsand. No description available Figure 1: Reverse engineering the dynamics of a complex system. ( a ) The dynamics of the system is captured by the unknown nonlinear dynamic equation (1), which we attempt to reconstruct from empirical observations. ( b ) The dynamic equation is composed of three functions M 0 ( x ), M 1 ( x ) and M 2 ( x ), defining the system’s model m as a point in the model space, . ( c , d ) To find this point we measure the system’s response to permanent perturbations, allowing us to extract a set of observable functions directly linked to m : ( c ) the transient response is characterized by the steady-state x i and the relaxation time τ i , from which we extract the exponents ξ and θ ; ( d ) the asymptotic response allows us to measure six additional functions (see Table 1 ), providing δ , ϕ , β , ω , σ and ν . ( e ) The eight functions of and allow us to infer the minimal subspace , which includes all potential models m that can describe the system’s dynamics. The dynamic equation in a is consistent with the observations in c and d if and only if . Full size image Traditionally, uncovering m involves three steps: (i) observation of the system’s macroscopic behaviour (ref. 17 ); (ii) inference of the microscopic model, m , from ; (iii) validation, showing that m can predict the observed behaviour . While this program has been successfully carried out for some well studied systems, the three steps above are difficult to replicate for complex systems: for instance, we lack general guidelines to choose the observation and a methodology to reliably translate it into a microscopic model. Hence steps (i) and (ii) require either an intuitive leap to guess the right observation and its inferred m , or exogenous knowledge, such as a mechanistic understanding of the nature of the interactions between the system’s components, knowledge we currently lack for many complex systems. Moreover, once m is found, step (iii) is insufficient to verify its uniqueness. Indeed, the inferred m could be one of a family of potential models that predict , which, absent any additional knowledge or observations, are all equally likely candidates for the system. This implies that rather than a specific point in the model space, what the observation truly allows us to infer is a broader subspace , comprising all models m that can be validated against . A model not included in can be ruled out by , however, all models that are included in this subspace are equally likely candidates and alone cannot be used to settle between them. Hence our goal is to develop a general method to infer , relying on minimal a priori knowledge of the structure of M 0 ( x ), M 1 ( x ) and M 2 ( x ). Our method provides a systematic formalism to treat all steps (i)–(iii) above for constructing m directly from empirical data. As our input observation we use the system’s response to external perturbations. This represents a common empirical exploration of complex systems, such as genetic perturbations in biology [18] , [19] , monitoring the impact of local failures in technological systems [20] or tracking the spread of information in social networks [21] , [22] . Our key result is linking the observed system response to the leading terms of m , providing a direct formulation by which to translate into an equation of the form (1). The inferred equation, reverse engineered directly from the data, does not provide a specific model m , but rather, defines the exact boundaries of , providing the most general class of dynamics that can be used to describe the observed system in light of . From observation to inference and validation To infer m we express its components in terms of a Hahn series [23] as which is a generalization of the Taylor expansion to include both negative and real powers. The powers Π i ( n ) represent a well-ordered set in ascending order with n , namely Π i (0) represents the leading power in the expansion of M i ( x ) around x 0 , Π i (1)>Π i (0) is the next power and so on. For certain systems the functional form of (3)–(5) is known, and the challenge is to infer the specific coefficients A n , B n and C n , which capture the model parameters, such as the rate constants in (1; refs 24 , 25 , 26 ). In contrast, here we consider systems whose microscopic model itself is unknown. Our goal is thus to uncover the functional form of (3)–(5), which is captured by the powers Π i ( n ) that participate in the expansion. Hence we do not focus here on distinctions such as M 2 ( x )= x 2 or M 2 ( x )=2 x 2 , a distinction regarding the coefficient C n , which describes the rate at which the interaction occurs. Rather, our focus here is on distinguishing between M 2 ( x ) ∼ x 2 versus, say, M 2 ( x ) ∼ 1– x −2 , as the different powers expressed in the expansion, Π 2 ( n ), capture different interaction mechanisms, and hence provide an insight into the fundamental characteristics of the system’s dynamics. To infer the leading powers of (3)–(5) we link them to a set of experimentally accessible observables, related to the system’s response to external perturbations. These observables, in turn, allow us to recover the structure of (3)–(5), reverse engineering the dynamics (1) to its leading terms. To conduct the observation, first we subject the nodes to external perturbations: this entails permanently perturbing the steady-state activity, x j of node j , and capturing the response of all other node activities x i ( t ). This could be achieved either through a controlled experiment, as frequently done in genetic perturbations [18] , or by monitoring natural perturbations, like observing the spread of ideas or memes in a social network [21] , [22] , or cascading failures in technological systems [20] . The impact of these perturbations is captured by two quantities (observations): Transient response . The temporal dynamics following a permanent perturbation is characterized by the time-dependent relaxation from the original steady state, x i , to the perturbed steady-state x i ( t →∞)= x i +d x i . By linearizing (1) around the steady state we find ( Supplementary Note 1 ) where τ i is node i ’s relaxation time and accounts for the propagation of the permanent perturbation along a distance l ij from the source j to the observed node i . Asymptotic response . After relaxation ( t ≫ max( τ i )), the system reaches a new, permanently perturbed state, captured by the response matrix [6] , [7] , [19] , [27] which quantifies the response of node i to j ’s perturbation ( Supplementary Note 2 ). By extracting a set of empirically observable exponents from the transient and the asymptotic responses, we can link x i ( t ) (6) and G ij (7) to m (2) via ( Supplementary Note 3 ) where and x 0 and y 0 are arbitrary constants. Equations (8)–(11), , ,  take a set of observables (exponents) extracted from the two observations, (6) and (7), as input (see Table 1 ), and provide the leading powers in the expansions (3)–(5) as output. From we can directly extract two exponents ( Supplementary Note 1 ): (i) θ captures the dependence of the relaxation time on the node’s degree k i , which follows the scaling and (ii) ξ describes the steady-state activity, which can either follow ( Supplementary Note 1 ) (scaling) or (saturation). From we can extract ( Supplementary Note 2 , ref. 7 ): (i) ϕ , capturing i ’s impact on its local neighbourhood , which scales as ; (ii) δ , capturing i ’s stability against perturbations in its vicinity , which follows ; and (iii) β , the dissipation rate that captures the behaviour of the distance-dependent propagation function, Γ( l ). This function describes the aggregated response of all nodes at distance l from a perturbation. For a system following (1) we have Γ( l )= e − βαl , where α =ln(〈 k 2 〉/〈 k 〉−1) is the expansion rate of the network. Note that to measure the observables used for the reconstruction (8)–(11) we must have access to the degrees k i of all the nodes, requiring us to know the network topology A ij . Later we show that even without access to A ij , a partial reconstruction of m is still possible. Table 1 Observations and . Full size table The inference presented in (8)–(11) provides only the leading terms of M 0 ( x ), M 1 ( x ) and M 2 ( x ). This leaves a degree of freedom to add additional terms, as denoted by , which involves all the terms of order higher (Θ + ( y )) or lower (Θ − ( y )) than x y . Finally, in (11) we used the unsigned Θ( y )=Θ sign( y ) ( y ), which allows the inclusion of higher (lower) powers for y>0 ( y<0 ). Hence by measuring the three characteristic exponents of ( δ , ϕ and β ), together with the two characteristic exponents of ( θ and ξ ), we can reconstruct m to its leading order terms, allowing us to write an effective continuum equation (1) for the system. Equations (8)–(11), , ,  represent our main result, offering a formalism to systematically reconstruct the dynamical equation governing a complex system. As expected, they do not point to a specific model, m , but narrow down the space of all the potential models into the minimal subspace of the models that are consistent with observations and ( Fig. 1e ). This subspace is robust to adding higher order terms and to parameter selection (that is, rate constants). Therefore it defines a minimal model, capturing the essential aspects of the mechanisms underlying the system’s interactions. Most importantly, our formalism guarantees that all models included in will successfully validate against and , and conversely all models for which will not be consistent with observations and . Hence if and only if can m be validated against the experimentally measured ξ and θ ( ), and δ , ϕ and β ( ). Inferring the dynamics of a model system To illustrate the predictive power of the developed formalism we first apply it to gene regulation, where the interaction is captured by a Hill function as (refs 13 , 14 , 28 ) Here B is a rate constant, a represents the level of self-regulation and the Hill coefficient, h , describes the level of cooperativity in gene regulation. We set B =1, a =1/2 and h =1/3, hence the real dynamics (12) is captured by the model Next we assume that m Real is unknown and preform an in silico reconstruction using (8)–(10). To observe and we perturb each node around the steady state and numerically measure x i ( t ) (6) and G ij (7) ( Supplementary Note 4 ). For we find ξ =2.0±0.02 and θ =1.0±0.01 ( Fig. 2a,b ); for we observe δ =0, ϕ =0.33±0.01 and β =0.67±0.01 ( Fig. 2c–e ). 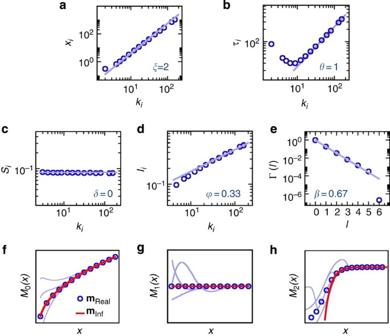Figure 2: Reverse-engineering regulatory dynamics. We constructed anin silicoregulatory network by numerically simulating regulatory dynamics (12) on a scale-free network,P(k)∼k−γ,γ=3, withN=6,000 nodes. Perturbing the activity of each node around its steady state, we measured the functions ofand. (a,b) Transient response: the steady-statexiscales withkiaswhereξ=2; the relaxation timeτihasθ=1. (c–e) Asymptotic response: fromGij(7) we measured the stabilitySi(δ=0), the impactIi(ϕ=0.33) and the propagation function Γ(l) (β=0.67). (f–h) Reverse engineered modelm: using equations (8)–(10), ,  we reverse engineered the dynamical equation obtaining the inferred model (14) (mInf, red solid lines). This model accurately recovers the leading terms of the original regulatory dynamics (13) (mReal, blue circles). As our formalism infers only the leading terms ofm, it allows for a degree of freedom to add additional terms, providing the minimal model subspaceof all the potential dynamics. Several functions from this subspace are also shown (violet solid lines). Note that all functions in the inferredaccurately capture the asymptotic behaviour of the real dynamics. Specifically, they correctly identify the essential feature of the regulatory dynamics, which is the saturation of the Hill function (M2(x)) for largex(h). Therefore (8)–(10) predict ( Supplementary Note 4 ) Figure 2: Reverse-engineering regulatory dynamics. We constructed an in silico regulatory network by numerically simulating regulatory dynamics (12) on a scale-free network, P ( k ) ∼ k − γ , γ =3, with N =6,000 nodes. Perturbing the activity of each node around its steady state, we measured the functions of and . ( a , b ) Transient response : the steady-state x i scales with k i as where ξ =2; the relaxation time τ i has θ =1. ( c – e ) Asymptotic response : from G ij (7) we measured the stability S i ( δ =0), the impact I i ( ϕ =0.33) and the propagation function Γ( l ) ( β =0.67). ( f – h ) Reverse engineered model m : using equations (8)–(10), ,  we reverse engineered the dynamical equation obtaining the inferred model (14) ( m Inf , red solid lines). This model accurately recovers the leading terms of the original regulatory dynamics (13) ( m Real , blue circles). As our formalism infers only the leading terms of m , it allows for a degree of freedom to add additional terms, providing the minimal model subspace of all the potential dynamics. Several functions from this subspace are also shown (violet solid lines). Note that all functions in the inferred accurately capture the asymptotic behaviour of the real dynamics. Specifically, they correctly identify the essential feature of the regulatory dynamics, which is the saturation of the Hill function ( M 2 ( x )) for large x ( h ). Full size image where η =0.50±0.01 and ρ =0.33±0.03. Hence the reverse engineered dynamical model for the system has the form where we only included the leading terms of (14). Equation (15) accurately recovers the self-dynamics and the interaction terms to leading order ( Fig. 2f–h ). Indeed, expanding M 2 ( x ) in (13) for large x leads to the inferred M 2 ( x ) in (15). Hence, the inferred M 2 ( x ) not only captures the qualitative form of the Hill function, that is, the saturation of the interaction term for large x (ref. 28 ), but also the precise form of that saturation as 1− x −1/3 +…. This demonstrates that our formalism can correctly reverse engineer the system’s microscopic dynamics directly from observing and . The inferred m can be also used to predict a broader range of macroscopic functions of direct experimental interest. Consider for example the probability density P ( G ) that a response term G ij is between G and G + dG . We can show that P ( G ) ∼ G − ν , where ν =( β +2)/( β +1) (ref. 7 ). Another quantity frequently observed in biological [18] , social [21] , [22] , [29] and technological [20] , [30] , [31] networks is the cascade size distribution, P ( C ), representing the probability that exactly C nodes exhibit a significant response (above a threshold) to a perturbation. This distribution is driven by the degree distribution through , where ω =( β + ϕ )/( β +1), predicting P ( C ) through P ( C ) ∼ P ( k ω = C ) (ref. 7 ). Finally, the incoming cascade of node i , defined as the group of all nodes whose perturbation impacted i above a threshold, can be shown to follow where σ =( β − δ )/( β +1). Hence, by recovering β , ϕ and δ , the inferred m is guaranteed to also predict P ( G ), P ( C ) and P ( Q ) ( Supplementary Note 2 ). Inferring the dynamics of empirical systems In experimental settings, we rarely have access to all the components of and . In some cases we may lack access to the temporal dynamics, unable to measure ξ and θ ; in others we lack a map of the underlying network, missing k i . Fortunately, the three additional exponents ν , ω and σ , associated with the cascades and with the distribution of terms in G ij ( Table 1 ), provide an excess of experimentally accessible quantities to arrive at the original exponents required for the reconstruction (8)–(10). This redundancy enables us to obtain insights from partial observations as well. We illustrate this by inferring the dynamical model for two systems that span rather different domains of inquiry: cell biology and human activity. Reverse-engineering subcellular dynamics. We demonstrate the utility of our formalism using results obtained from high-throughput gene perturbation experiments for S. cerevisiae . Here G ij measures the change in the expression levels of 6,222 yeast genes induced by 55 individual genetic perturbations [32] . As the data set is not time resolved, we lack access to . We also lack an accurate map of the underlying regulatory/protein interaction network, hence we cannot directly measure δ , ϕ and β . Our method offers valuable insights even under these rather limiting circumstances. First, we measure the distribution of terms in G ij , which we find to follow P ( G ) ∼ G − ν where ν =2.0±0.1 ( Fig. 3a ). Using Table 1 this translates to β =0. Next we measure the distribution P ( Q ) of the incoming cascades of all the nodes ( Fig. 3b ). Its bounded nature implies that it is disconnected from the degree heterogeneity ( P ( k )) [33] , [34] , possible only if σ =0, which in turn provides δ =0 ( Table 1 ). 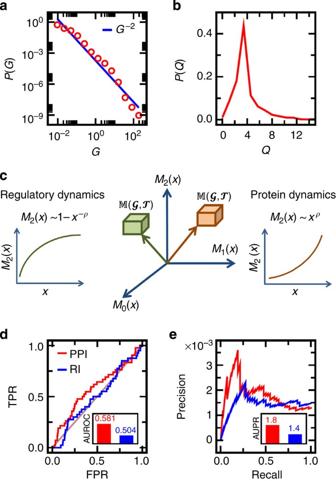Figure 3: Reverse-engineering subcellular dynamics. We constructedGijfrom high-throughput microarray data tracking the response of 6,222 target genes to the perturbation of 55 transcription factors in yeast32. (a) The response distribution is well approximated with a power lawP(G)∼G−νwith exponentν=2. UsingTable 1this predictsβ=0. (b) The incoming cascade size distribution,P(Q), is bounded (seeSupplementary Note 6), indicating thatQiis independent ofki; consequentlyσ=0, predicting alsoδ=0 (Table 1). (c) As here we only have access to two functions from the observationand no access toa all, the model subspace,, that we infer includes a broad range of potential models, as indicated by the nonspecific form of (16). Still, the inferred model can help us distinguish between two competing processes in cellular dynamics, which occupy distinct areas in the model space: RIs are characterized byM2(x), which saturates for largex(activation/inhibition13,14); protein–protein interactions are captured by a non-saturating polynomialM2(x) (mass action8,9). The inferred model (16), withM2(x)∼xρ, belongs to the protein interaction class of dynamics. (d,e) We usedGijto predict PPIs (red) and RIs (blue), and measured AUROC and AUPR to evaluate the performance of the two predictions. For RIs we have AUROC=0.504 and AUPR=1.4 × 10−3, indistinguishable from a random guess (Supplementary Note 6). For protein interactions we have AUROC=0.580 and AUPR=1.8 × 10−3(Pvalues 0.03 and 0.07), indicating that indeed, the observedGijis a better predictor of protein interactions than of RIs (TPR, true positive rate; FPR, false positive rate). Hence using (8)–(10) we obtain ( Supplementary Note 6 ) Figure 3: Reverse-engineering subcellular dynamics. We constructed G ij from high-throughput microarray data tracking the response of 6,222 target genes to the perturbation of 55 transcription factors in yeast [32] . ( a ) The response distribution is well approximated with a power law P ( G ) ∼ G − ν with exponent ν =2. Using Table 1 this predicts β =0. ( b ) The incoming cascade size distribution, P ( Q ), is bounded (see Supplementary Note 6 ), indicating that Q i is independent of k i ; consequently σ =0, predicting also δ =0 ( Table 1 ). ( c ) As here we only have access to two functions from the observation and no access to a all, the model subspace, , that we infer includes a broad range of potential models, as indicated by the nonspecific form of (16). Still, the inferred model can help us distinguish between two competing processes in cellular dynamics, which occupy distinct areas in the model space : RIs are characterized by M 2 ( x ), which saturates for large x (activation/inhibition [13] , [14] ); protein–protein interactions are captured by a non-saturating polynomial M 2 ( x ) (mass action [8] , [9] ). The inferred model (16), with M 2 ( x ) ∼ x ρ , belongs to the protein interaction class of dynamics. ( d , e ) We used G ij to predict PPIs (red) and RIs (blue), and measured AUROC and AUPR to evaluate the performance of the two predictions. For RIs we have AUROC=0.504 and AUPR=1.4 × 10 −3 , indistinguishable from a random guess ( Supplementary Note 6 ). For protein interactions we have AUROC=0.580 and AUPR=1.8 × 10 −3 ( P values 0.03 and 0.07), indicating that indeed, the observed G ij is a better predictor of protein interactions than of RIs (TPR, true positive rate; FPR, false positive rate). Full size image where, for simplicity, we once again omitted the higher order terms. Equation (16) predicts a family of potential models, with an arbitrary M 1 ( x ) and η and ρ , degrees of freedom originating in our partial coverage of the functions used as input in (8)–(10). Indeed, it is expected than the less specific is the observation , the broader are the limits of the inferred subspace . Despite these degrees of freedom, (16) offers crucial insight into the biological mechanisms that underlie the observed dynamics, helping us distinguish between the two classes of dynamical processes that potentially drive the expression patterns of genes in the studied experiment. The first process is regulatory interactions (RIs), the mutual activation/inhibition of genes, in which the interaction term has the form of a switch-like function, for example, Hill function (12), saturating as M 2 ( x →∞)→1 ( M 2 ( x →∞)→0), to describe the activation (inhibition) [13] , [14] ( Figs 2h and 3c ). A competing process is protein–protein interactions (PPIs), a biochemical mechanism in which proteins physically bind to each other. PPIs are expressed in (1) through mass action kinetics by non-saturating polynomial terms. Indeed, according to the law of mass action a physical binding interaction μA + ρB → AB contributes a term of the form to the relevant equations in (1) (refs 9 , 15 , 35 , 36 ). Hence the polynomial (non-saturating) form of M 0 ( x ) and M 2 ( x ) in (16) indicates that in this experiment the system’s dynamics is dominated by biochemical interactions, such as protein binding, degradation and dimerization, rather than genetic regulation. To directly test this prediction we used validated lists of 2,930 PPIs (ref. 34 ) and 1,079 RIs [37] . It is expected that a large response G ij indicates an increased probability of finding a direct i, j link. Hence we can use G ij to predict the already known PPI/RI links. The standard measures to evaluate such predictions are the areas under the receiver operating curve (AUROC) and under the precision recall curve (AUPR) [38] ( Supplementary Note 6 ). Measuring these curves ( Fig. 3d,e ), we find that in this experiment G ij is indeed more predictive of PPIs than of RIs: for PPIs we obtain AUROC=0.580 ( P value 0.03, Supplementary Note 6 ) and AUPR=1.8 × 10 −3 ( P value 0.07), while for RIs we find AUROC=0.504, and AUPR=1.4 × 10 −3 , both not significantly better than random ( P value ∼ 1). Hence, even though cellular dynamics is driven by a combinations of both RIs and PPIs, in this experiment G ij emphasizes PPIs significantly more than the RIs, supporting our conclusion that PPIs, driven by biochemistry, offer the dominant contribution to the experimentally observed G ij , in agreement with the inferred (16). This finding is, in fact, consistent with other studies indicating that PPIs play a significant role in shaping the profile of expression data [39] , [40] , [41] . Therefore the strength of our formalism is not only its ability to reconstruct the continuum model (16), but also its ability to detect the dominance of PPIs in this experiment using only the observed data G ij . Reverse-engineering human dynamics. While building continuum models for biological systems has a long tradition, the diversity of human interaction has lead to a paucity of continuum models capturing human dynamics [42] , [43] . Here we rely on a data set that captures ∼ 6 × 10 4 exchanges between 1,899 users of an online instant messaging service (UCIonline) during a ∼ 7 month period (ref. 44 ). This allowed us to construct A ij by linking each user pair that exchanged at least one message during the documented period. As here we cannot conduct a controlled perturbation experiment, we rely on proxies that capture quantities associated with x i in (6) and G ij in (7). First we measure the number of messages sent by user i during a 3 hours interval, x i ( t ), to obtain its time-dependent activity. We take x i =< x i ( t )> as a proxy for i ’s steady-state activity and as a proxy for (7) ( Supplementary Note 7 ). We find ξ =1.23±0.03, δ =0 and ν =1.60±0.03, predicting β =0.67 ( Table 1 , Fig. 4a–c ). 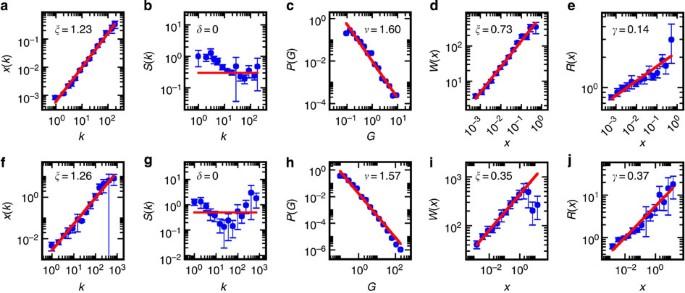Figure 4: Reverse-engineering human dynamics. As a proxy for human dynamics we used data on the activity patterns of 1,899 individuals who exchanged messages in an online social network (UCIonline44). (a) Using the average activity (messages per unit time) of a node as a proxy forxiwe obtainξ=1.23. (b) The stability does not scale withki, indicating thatδ=0. (c) The response distributionP(G) is well approximated with a power law withν=1.60, predictingβ=0.67 (Table 1). (d) We approximate the workloadWiof useriby measuring its incoming messages, finding thatwithζ=0.73. (e) The responsiveness,Ri, denoting the ratio of outgoing to incoming messages ini’s account is found to scale as, withγ=0.14. (f–h) We measured the exponentsξ,δandνfrom an independent email data set (Epoch45), finding that the two systems feature similar behaviour. (i) The workload, however, differs across the two data sets withζ=0.35, predicting that in the the reverse engineered equation (18) the exponentμis greater in Epoch than in UCIonline. (j) As a consequence (18) predicts a stronger dependence betweenRiandxifor email communications compared with online messaging. Indeed we find that for Epochγ=0.37, greater than the value observed for UCIonline (0.14). This correct prediction of (18) provides independent support for its validity. All error bars represent 95% confidence intervals (Supplementary Note 4). Hence equations (8)–(10), ,  predict that the continuum model capturing the dynamics of this social system has the form Figure 4: Reverse-engineering human dynamics. As a proxy for human dynamics we used data on the activity patterns of 1,899 individuals who exchanged messages in an online social network (UCIonline [44] ). ( a ) Using the average activity (messages per unit time) of a node as a proxy for x i we obtain ξ =1.23. ( b ) The stability does not scale with k i , indicating that δ =0. ( c ) The response distribution P ( G ) is well approximated with a power law with ν =1.60, predicting β =0.67 ( Table 1 ). ( d ) We approximate the workload W i of user i by measuring its incoming messages, finding that with ζ =0.73. ( e ) The responsiveness, R i , denoting the ratio of outgoing to incoming messages in i ’s account is found to scale as , with γ =0.14. ( f – h ) We measured the exponents ξ , δ and ν from an independent email data set (Epoch [45] ), finding that the two systems feature similar behaviour. ( i ) The workload, however, differs across the two data sets with ζ =0.35, predicting that in the the reverse engineered equation (18) the exponent μ is greater in Epoch than in UCIonline. ( j ) As a consequence (18) predicts a stronger dependence between R i and x i for email communications compared with online messaging. Indeed we find that for Epoch γ =0.37, greater than the value observed for UCIonline (0.14). This correct prediction of (18) provides independent support for its validity. All error bars represent 95% confidence intervals ( Supplementary Note 4 ). Full size image where η =0.81, ρ =0.54 and M 1 ( x ) is an arbitrary function. To understand the inferred dynamics, we expand M 1 ( x i ) as in (4) and take its leading power to be μ , namely Π 1 (0)= μ . Hence the self-dynamic term in (17) becomes . Note that this term provides the node’s dynamics in isolation, as in the absence of interacting partners equation (1) reduces to . Here as we describe the message exchanges between linked individuals, an isolated node should become inactive, x i ( t →∞)=0, a condition satisfied if we set x 0 =0. Hence, taking only the leading terms of m Human we obtain the continuum equation To evaluate μ we consider the workload W i of pending messages that have to be sent or replied and its impact on i ’s activity x i . When the workload W i is large, i experiences a significant pressure to respond, increasing its activity x i . Yet W i decreases with every email i sends, hence a highly active i will rapidly decrease its workload and activity. Equation (18) predicts that the workload should increase with i ’s activity as ( Supplementary Note 7 ) where ζ =2– η – μ . To test the validity of this prediction we measured the incoming messages of all nodes as a proxy for their workload, finding that the predicted scaling (19) holds for over three orders of magnitude with ζ =0.73±0.02, predicting μ =0.46 ( Fig. 4d ). The second term on the right hand side of equation (18) describes the impact of the neighbours’ activity x j on x i . An active neighbour j increases i ’s activity, prompting it to reply or forward its incoming messages. The saturating nature of M 2 ( x ), however, indicates that a neighbour’s impact is bounded, reaching a maximum of y 0 . This agrees with our expectation that even an extremely active neighbour cannot drive its contacts to be active beyond their maximal capacity. To validate (18) we used an independent data set, recording ∼ 3 × 10 5 email exchanges between 2,688 users during a ∼ 6-month period (Epoch) (ref. 45 ). The exponents extracted from this data set are very close to those obtained from UCIonline: ξ =1.26±0.04, δ =0 and ν =1.57±0.05 ( Fig. 4f–h ). The workload (19), however, has ζ =0.35±0.1, which significantly differs from that of UCIonline ( Fig. 4i ). Reverse engineering the dynamics from these exponents leads to (18), with η =0.79, μ =0.86 and ρ =0.60. This striking agreement between the structure of the two equations inferred from two independent data sets, indicates that the reverse engineered (18) captures the fundamental dynamical characteristics of human communications. The only notable difference between the two inferred models is in the value of μ , which is higher in Epoch than in UCIonline. This parameter characterizes the correlation between a node’s activity and its tendency to respond to incoming messages ( Supplementary Note 7 ). Hence the greater value of μ in Epoch suggests that the propensity to respond to incoming communications is more strongly dependent on the activity in email communication than in instant messaging. To test if this is indeed the case we measured the responsiveness, R i , of all nodes, defined as the average ratio between the incoming and outgoing traffic between i and its interacting partners. As μ is greater for Epoch than UCIonline, we expect a stronger dependency in Epoch between R i and x i than in UCIonline. Indeed, as shown in Fig. 4e,j this prediction is valid: the scaling of R i with x i , is greater for Epoch ( γ =0.37) than for UCIonline ( γ =0.14). This dynamical distinction, correctly predicted by the reverse engineered equations, provides independent support for the predictive power of our formalism. The empirical results presented above demonstrate the practical applicability of our methodology, which is a result of the robust nature of its underlying observables. Indeed, characteristic exponents and scaling laws, the basis of our reverse-engineering formalism, are often universal [46] , and hence unaffected by the microscopic details of the system’s topology and dynamics [7] . This allows us to reliably measure the observables even for real systems, which rarely satisfy all of the model assumptions, for example, they are subject to the effect of noise, both in their dynamics as well as in their topology. For example, many real networks feature degree correlations, which, strictly speaking, violate our formalism’s predictions ( Supplementary Note 1 ). Fortunately, the observed exponents are rather insensitive to such microscopic discrepancies, and can be accurately extracted from both model and empirical systems, even in the presence of degree correlations. To exemplify this we simulated the predicted human dynamics (18) on the empirical network of Email Epoch. Even though this network features rather strong degree correlations, we show in Supplementary Note 7 that the measured obsevables, that is, the exponents ξ , δ and ν , can be accurately fitted by the predictions of our formalism. In summary, the technological and experimental advances of recent years have offered a wealth of data, capturing the detailed node-level dynamics of biological, social and technological systems. It is difficult, however, to extract predictive power of these systems without a mechanistic model. Such models are rare for complex systems, however. Here we address this challenge as a reverse-engineering problem, showing that we can use the data to peek into the inner mechanisms of the system, providing an analytical microscope into the dynamics of a complex system. We tested our formalism under rather strict conditions, inferring m from scratch, relying only on the system’s macroscopic behaviour ( and ). A more realistic scenario, however, is to use the proposed method in conjunction with some prior knowledge about the system’s microscopic dynamics. Often we seek a resolution between two or more competing models, as was the case in our inference of the cellular dynamics. If the two candidate models have a different functional form in (1), they will occupy distinct subspaces in , and the more likely of the two can be decisively determined ( Fig. 3c ). In other cases, the inference can be supported by some a priori knowledge pertaining to the system’s behaviour. For instance, in human dynamics we postulated, based on the nature of the observed system, that isolated individuals should become inactive. Coupled with our formalism (8)–(10), this allowed us to complete the reconstruction of (18). Other practical considerations in reverse engineering are addressed in Supplementary Note 7 . Finally, the fact that our formalism infers a subspace , rather than a specific model m provides us with exact bounds on the predictive power of an observation. Indeed, it tells us that our observation, , provides us with theoretical grounds to select over . At the same time, however, our formalism shows that cannot be used to discriminate between any set of models within , by that marking the theoretical limits on the specificity of the inferred model. How to cite this article: Barzel, B. et al . Constructing minimal models for complex system dynamics. Nat. Commun. 6:7186 doi: 10.1038/ncomms8186 (2015).